Universal passivation strategy to slot-die printed SnO2for hysteresis-free efficient flexible perovskite solar module Perovskite solar cells (PSCs) have reached an impressive efficiency over 23%. One of its promising characteristics is the low-cost solution printability, especially for flexible solar cells. However, printing large area uniform electron transport layers on rough and soft plastic substrates without hysteresis is still a great challenge. Herein, we demonstrate slot-die printed high quality tin oxide films for high efficiency flexible PSCs. The inherent hysteresis induced by the tin oxide layer is suppressed using a universal potassium interfacial passivation strategy regardless of fabricating methods. Results show that the potassium cations, not the anions, facilitate the growth of perovskite grains, passivate the interface, and contribute to the enhanced efficiency and stability. The small size flexible PSCs achieve a high efficiency of 17.18% and large size (5 × 6 cm 2 ) flexible modules obtain an efficiency over 15%. This passivation strategy has shown great promise for pursuing high performance large area flexible PSCs. Organic–inorganic metal halide perovskite solar cells (PSCs) have shown promising for commercial applications due to its low-cost and high power conversion efficiency (PCE) [1] , [2] , [3] , [4] , [5] . Recently, the planar structured PSCs have attracted increasing interest because of its simple structure and easy fabrication [6] , [7] . To improve the performance of the planar PSCs, the bottom electron transport layer (ETL) is extremely important. It should be transparent for visible light, photo-stable and compatible with the perovskites. The SnO 2 has shown a good candidate for the efficient and stable ETL [7] , [8] , [9] . It can be fabricated via a low-temperature process and suitable for the flexible PSCs that possess light-weight, low-cost, weak-light photovoltaic and flexibility [10] , [11] . This opens possible alternative applications, such as portable power source for wearable electronics and energy source for indoor sensors. More importantly, for some special applications, such as indoor sensors, the requirement of the PCE and stability would be less demanding compared with the roof solar panels. Thus, it could accelerate commercial applications of the PSCs. Aiming for the commercialization, fabrication of large-area PSC modules (PSCMs) has been becoming the focus of research. Although the flexible PSCs have been widely studied, the PCE of flexible PSCMs is still quite low, only 8% reported by Dagar et al. and others [12] , [13] . To achieve an efficient planar flexible PSC, besides the quality control of the perovskites, the charge extraction layer underneath the perovskite is more difficult to fabricate compared with that on the glass substrate. The ETL is quite thin with the thickness varying from a few nm to tens of nm. To fabricate large-area thin-film ETL without pinholes on the rough and flexible plastic substrate is of great challenge [14] . In addition, devices on plastic substrates generally limit the processing temperature below ~150 °C. Furthermore, the perovskite/ETL or HTL interfaces have been considered as serious problems which are relevant to the defects and imbalanced charge transport leading to poor performance, instability and hysteresis [15] , [16] , [17] , [18] , [19] . SnO 2 ETLs can be fabricated via various methods at low temperature, including spin-coating, chemical bath deposition (CBD), atomic-layer deposition (ALD), etc. for planar PSCs [7] , [8] , [9] , [11] , [20] , [21] , [22] , [23] , [24] . It has been well accepted that the SnO 2 could benefit the elimination of the hysteresis, a common issue in TiO 2 ETL-based PSCs since the SnO 2 has a deeper conduction band edge and a faster electron mobility than the TiO 2 [7] , [9] . Hysteresis-free devices have indeed been fabricated by several groups using a commercial SnO 2 colloid precursor (Alfa Aesar, tin (IV) oxide, 15% in H 2 O colloidal dispersion, labelled as Alfa–SnO 2 ) [7] . 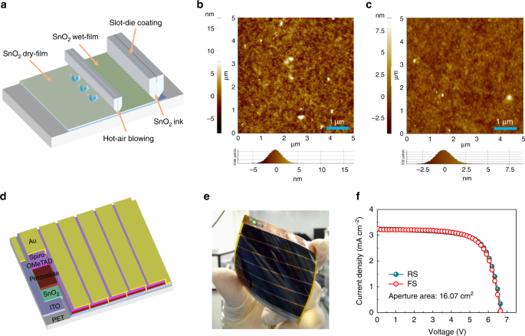Fig. 1 Performance of large-area flexible PSCMs based on slot-die-coated SnO2substrates.aThe schematic of slot-die coating of SnO2films.bAFM images of the as formed SnO2films without hot air assistance andcwith hot air blowing.dThe structure of the 6 sections series connected large-area flexible PSCMs.eA photograph of the flexible PSCM andfthe correspondingJ-Vcurves of the champion flexible PSCM However, as the hysteresis is not only related to the charge extraction at the interface, more and more reports have shown the hysteresis still presented in the SnO 2 -based planar PSCs if without additional interfacial treatment (Supplementary Table 1 ) [9] , [10] , [20] , [25] , [26] , [27] , [28] , [29] , [30] . The intrinsic reason why the low-temperature processed Alfa–SnO 2 ETL can eliminate the hysteresis is still unclear. Here, we investigate the Alfa–SnO 2 in detail and find that in the Alfa–SnO 2 colloid solution there was potassium hydroxide (KOH) added to stabilize the colloids. The crucial effect of hysteresis is ascribed to the interface passivation induced by the potassium ions. Then we employ this Alfa–SnO 2 to fabricate flexible PSCMs. By optimization of the slot-die coating of this Alfa–SnO 2 colloid solution onto the flexible ITO/PET substrate, combining with the modulation of mixed lead halide perovskite cations, such as methylammonium (CH 3 NH 3 + , MA), formamidinium (CH 3 (NH 2 ) 2 + , FA) and cesium (Cs), we obtain a 5 × 6 cm 2 large area (aperture area of 16.07 cm 2 ) flexible PSCM with high efficiency over 15% and negligible hysteresis. The Alfa–SnO 2 has showed good performance as effective ETLs. However, considering the strong basicity (pH value is ~12) of the commercial Alfa–SnO 2 solution, it is not suitable for production due to the alkali etching. Alternatively, we apply KOH onto the slot-die-coated the homemade SnO 2 nanocrystals (SnO 2 NCs) films [23] , since the potassium passivation effect could be a universal strategy to eliminate the hysteresis in the SnO 2 -based planar PSCs. A hysteresis-free high PCE of 20.50% for reverse scan (RS) and 20.46% for forward scan (FS) is obtained for rigid PSC, with dramatically improved V oc and FF compared with the control devices which show lower PCEs of 19.27% for RS and 16.42% for FS. In addition, the small size flexible PSCs and large size flexible PSCMs also show negligible hysteresis and achieved high PCEs of 17.18% for 0.16 cm 2 and 14.89% for 16.07 cm 2 . High efficiency flexible PSCMs based on Alfa–SnO 2 ETL Slot-die coating deposition is an excellent method for large-area mass production of solution-processed films, but the solution used for the slot-die coating should be carefully adjusted, such as viscosity, volatility, wettability, toxicity, etc. Herein, the as-purchased Alfa–SnO 2 colloidal dispersion in water was first diluted by water and then by isopropanol drop by drop, and it was then slot-die-coated onto large-area (5 × 6 cm 2 ) flexible ITO/PET substrates as shown in Fig. 1a . A wind knife with hot air was attached to the slot-die head allowing the fast drying of the printed wet SnO 2 films on ITO/PET substrates, to prevent SnO 2 nanocrystals from aggregation in wet films, which would lead to a rough surface and pinholes in SnO 2 films. As demonstrated in Atomic Force Microscope (AFM) images (Fig. 1b, c ), the slot-die-coated SnO 2 films quickly dried by the hot air blowing showed a smooth and compact surface with a much lower roughness (0.95 nm) compared with the naturally dried films (5.3 nm). To evaluate the homogeneity of the coating technique, an as coated 5 × 6 cm 2 SnO 2 /ITO/PET substrate was equally cut into six pieces to measure the transmittance of SnO 2 films (Supplementary Fig. 1a ) under 550 nm light. The variation in the absorption at 550 nm was just only 3%, indicating that the film is highly uniform in such a large area. We also demonstrated the uniformity in microstructure (Supplementary Fig. 1b, c ), where the SEM images show pinhole-free morphology of the SnO 2 films deposited on the ITO/PET substrates. In addition, the transmittance of the substrates also showed an enhancement with coated SnO 2 films due to the reduced anti-reflection. Fig. 1 Performance of large-area flexible PSCMs based on slot-die-coated SnO 2 substrates. a The schematic of slot-die coating of SnO 2 films. b AFM images of the as formed SnO 2 films without hot air assistance and c with hot air blowing. d The structure of the 6 sections series connected large-area flexible PSCMs. e A photograph of the flexible PSCM and f the corresponding J-V curves of the champion flexible PSCM Full size image The perovskite composition selected for this study was Cs 0.05 (FA 0.85 MA 0.15 ) 0.95 Pb(I 0.85 Br 0.15 ) 3 . Perovskite films were spun onto the hot-air-assisted slot-die-coated large-area pinhole-free and high-quality SnO 2 /ITO/PET substrates via a green solvent engineering method [31] , and then the whole flexible PSCMs fabrication was accomplished according to our previous report [29] . The structure of the PSCMs are illustrated in Fig. 1d , which are series connected by six subcells. And each cell is in a structure of PET/ITO/SnO 2 /perovskite/Spiro-OMeTAD/Au, respectively. Interestingly, the as-prepared flexible PSCM could light up a green LED lamp even in an indoor light, as shown in Fig. 1e , revealing its excellent photovoltaic property under weak light. The corresponding J-V curves of the champion PSCM are shown in Fig. 1f , with a high PCE of 15.22% for reverse scan (RS) and 15.10% for forward scan (RS), and a high V oc of 6.727 V for RS and 6.663 V for FS, a J sc of 3.28 mA cm −2 for RS and 3.28 mA cm −2 for FS, and a FF of 0.69 for RS and 0.69 for FS, respectively. The flexible module also exhibited outstanding stability which still remains 80% of its original efficiency after 1000 h dark storage in ambient air (~20% RH) without encapsulation (Supplementary Fig. 1d ). In addition, the bending stability is also an important parameter for evaluation of the performance of the flexible devices. Herein, the slot-die-coated SnO 2 -based flexible module showed superior resistance for the mechanical bending, with no more than 30% loss even after 1800 bending cycles (Supplementary Fig. 1e ). The main loss of the device performance after bending is the result of the increased FF caused by the increased R s (Supplementary Fig. 1f ) that is induced by the mechanical damage of the ITO conduction layer. This indicates that the great durability of the SnO 2 nanoparticles composed thin films are suitable for future industrial applications of flexible PSCMs. Intrinsic reason for Alfa–SnO 2 to eliminate hysteresis The hysteresis has been regarded as a serious problem in a normal planar PSC, due to its detrimental effect on the device performance and stability [15] , [32] , [33] , [34] . There are lots of reports described various types of SnO 2 ETLs formed by different synthesis methods, deposition ways and optimization techniques, and almost all of them presented non-negligible hysteresis [9] , [11] , [26] , [35] . However, the PSCMs prepared from the low-temperature deposited commercial Alfa–SnO 2 film in this work exhibited negligible hysteresis [7] . It is obviously interesting to find out the intrinsic reason for it. When carefully analysed the commercial Alfa–SnO 2 solution, we found that the Alfa–SnO 2 aqueous solution showed a strong basicity (pH ~12). Further investigation by the scanning transmission electron microscopy and energy dispersive X-ray spectroscopy (STEM–EDX) analysis revealed the presence of the K ions in the solution. The EDX mapping images (Fig. 2a ) of the polycrystalline Alfa–SnO 2 nanoparticles and the corresponding EDX images (Supplementary Fig. 2 ) of Sn, O and K elements, respectively, clearly demonstrate the existence of potassium ions. From the STEM–EDX elemental analysis, we further observed a K-rich phase located in a blank area compared with the SnO 2 nanoparticles rich areas (Fig. 2b ), which indicates that the potassium ions are mainly dissolved in the water not the SnO 2 nanocrystals. Thus, we conclude that the potassium hydroxide (KOH) was added in the solution as a stabilizer for the SnO 2 nanocrystals during this commercial Alfa–SnO 2 solution preparation. Recently, potassium ions have been added into perovskite and have shown efficient passivation effect to eliminate the hysteresis [29] , [36] . Therefore, the hysteresis elimination effect by this Alfa–SnO 2 should mainly be attributed to the passivation of potassium ions between the interface of SnO 2 and perovskite. Fig. 2 Characterization of the Alfa–SnO 2 and corresponding performance of PSCs. a The STEM–EDX images of the Alfa–SnO 2 colloidal. b The corresponding EDX spectra consistent to the boxed area. c The normalized SIMS results of the CsFAMA perovskite deposited on Alfa–SnO 2 /FTO substrate. d The XPS spectra of K2 p orbital of the pristine Alfa–SnO 2 films and Water Alfa–SnO 2 films. e The SEM images of Alfa–SnO 2 based CsFAMA perovskite film, f Water Alfa–SnO 2 -based CsFAMA perovskite film and g KOH-treated Water Alfa–SnO 2 -based CsFAMA perovskite film. h The J-V curves of Alfa–SnO 2 -based PSC, i Water Alfa–SnO 2 -based PSC and j KOH-treated Water Alfa–SnO 2 -based PSC, respectively Full size image To locate the distribution of the K ions, time of flight secondary ion mass spectrometry (TOF-SIMS) measurements were employed. 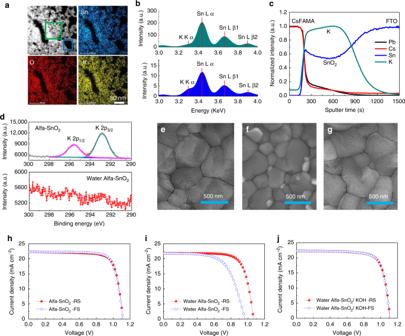Fig. 2 Characterization of the Alfa–SnO2and corresponding performance of PSCs.aThe STEM–EDX images of the Alfa–SnO2colloidal.bThe corresponding EDX spectra consistent to the boxed area.cThe normalized SIMS results of the CsFAMA perovskite deposited on Alfa–SnO2/FTO substrate.dThe XPS spectra of K2porbital of the pristine Alfa–SnO2films and Water Alfa–SnO2films.eThe SEM images of Alfa–SnO2based CsFAMA perovskite film,fWater Alfa–SnO2-based CsFAMA perovskite film andgKOH-treated Water Alfa–SnO2-based CsFAMA perovskite film.hTheJ-Vcurves of Alfa–SnO2-based PSC,iWater Alfa–SnO2-based PSC andjKOH-treated Water Alfa–SnO2-based PSC, respectively Figure 2c shows the normalized SIMS data of a CsFAMA film deposited on the Alfa–SnO 2 film, which reveals that potassium ions mainly remained in the SnO 2 ETL and at the interface between SnO 2 ETL and perovskite absorber layer. To further confirm the effect of the K ions, we use deionized water to bath the as-sintered Alfa–SnO 2 films to remove the residual potassium ions (labelled as Water Alfa–SnO 2 ). From the X-ray photoelectron spectroscopy (XPS) spectrum analysis, an outstanding peak of K2 p orbital was appeared in the pristine Alfa–SnO 2 films, while it disappeared after bathing for only10 min (Fig. 2d and Supplementary Fig. 3 ). This clearly indicates that the potassium ions are just blended with SnO 2 crystals and not doped into SnO 2 crystal lattices even after sintered at 150 °C. When the water washed SnO 2 ETL was made into devices, as predicted it showed a severe hysteresis due to the removal of the potassium in the Alfa–SnO 2 film, as well as a decreased performance from 19.06% for RS and 19.10% for FS to 17.40% for RS and 14.28% for FS (Fig. 2h, i ). However, when the Water Alfa–SnO 2 ETLs were re-treated with a KOH aqueous solution (10 mM, pH 12), which is labelled as the Water Alfa–SnO 2 /KOH, to introduce K ions back, the enhanced PCEs of 18.62% for RS and 18.57% for FS have been achieved with negligible hysteresis (Fig. 2j ). The detailed parameters are showed in Supplementary Table 2 . Actually, the perovskites deposited on the Alfa–SnO 2 ETL and Water Alfa–SnO 2 /KOH ETL have quite similar properties, including morphology, grain size (Fig. 2e–g ), XRD patterns, and UV-Vis Spectra, and corresponding EQE of devices, which are different with the perovskite deposited on the Water Alfa–SnO 2 ETL as shown in Supplementary Fig. 4 . This further confirmed the important role of the K ions at the interface on the performance of the planar PSCs, especially the hysteresis, which will be discussed in more details in the following parts. Potassium interface engineering for SnO 2 -based PSCs Based on above analysis, the potassium ions at the interface would benefit the planar PSCs not only for PCEs but also the hysteresis due to the passivation effect. As discussed, the reported SnO 2 ETLs synthesized via various methods without surface treatments almost all have the hysteresis issue. We thus treated different low-temperature processed SnO 2 films with the KOH aqueous solution to investigate the universality of this interface passivation strategy. In addition, we also aim to replace the strong alkaline Alfa–SnO 2 colloidal dispersion due to its disadvantages, such as strong corrosion to slot-die metal surface and poor wettability to plastic substrates (Supplementary Fig. 5 ). 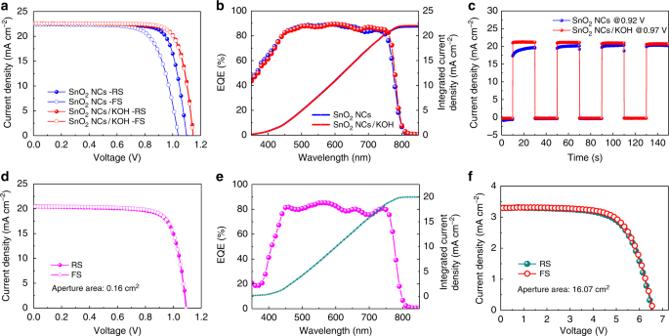Fig. 3 Performance of PSCs with interface potassium passivation.aThe championJ-Vcurves of SnO2NCs-based PSCs with potassium passivation or not.bThe corresponding EQE spectra of these champion devices.cSteady-state output current under maximum power point with regularly turn on/off test.dThe championJ-Vcurves of SnO2NCs-based flexible PSC with potassium passivation.eThe corresponding EQE spectra of this champion flexible device andftheJ-Vcurves of SnO2NCs-based large-area flexible PSCM Figure 3a shows the champion J-V curves of the low-temperature presynthesized highly crystalline SnO 2 nanocrystals (labelled as SnO 2 NCs) based PSCs with or without KOH treatment. The as-synthesized SnO 2 NCs are quite similar to Alfa–SnO 2 , with high crystallinity and negligible Cl − residuals (Supplementary Figs. 2 , 6 ). The corresponding performance of the devices treated with different concentrations of KOH solutions is shown in Supplementary Fig. 7 , and the detailed J-V parameters are illustrated in Supplementary Table 3 . The pristine device exhibits a typical J-V hysteresis, with a poor PCE of 16.42% under FS compared with the PCE of 19.27% under RS. When introducing an interface treatment of potassium ions by a 10 mM KOH solution treatment, an outstanding improvement of performance was obtained with a hysteresis-free high efficiency of 20.50% for RS and 20.46% for FS. The detailed parameters derived from the J-V curves are showed in Table 1 , and a mathematical statistical distribution of these devices are also exhibited in Supplementary Fig. 8 . It presents an obvious enhancement of V oc compared with the pristine devices, which indicates the slower charge carrier recombination at the interface of PSCs. Figure 3b shows the corresponding EQE spectra of these champion devices with an integrated current density of 21.78 mA cm −2 for pristine devices and 21.97 mA cm −2 for passivated devices, respectively, which are highly consistent to the J-V results. In addition, the photoelectric response of passivated device based on the turn on/off test for the output current measurement under the maximum power point is showed in Fig. 3c , which is much swifter than pristine devices. Moreover, these two devices were tested under AM 1.5 G continuously for five times. It is found that the potassium passivated device showed excellent light stability compared with the non-passivated device (Supplementary Fig. 9a, b ). The long-term stability of the passivated device is also much better than the non-passivated device, which decreased no more than 5% in its efficiency after 30 days when stored under dark in ambient air without encapsulation (Supplementary Fig. 9c ). Besides, the widely used chemical bath deposited SnO 2 films (labelled as CBD–SnO 2 ), spin-coated SnCl 4 /isopropanol solution (labelled as Spin-SnCl 4 ) with KOH treatment are also showed in Supplementary Fig. 10 , and both of them exhibit negligible hysteresis and improved performance, indicating a universal passivation for different SnO 2 substrate-based PSCs. Fig. 3 Performance of PSCs with interface potassium passivation. a The champion J-V curves of SnO 2 NCs-based PSCs with potassium passivation or not. b The corresponding EQE spectra of these champion devices. c Steady-state output current under maximum power point with regularly turn on/off test. d The champion J-V curves of SnO 2 NCs-based flexible PSC with potassium passivation. e The corresponding EQE spectra of this champion flexible device and f the J-V curves of SnO 2 NCs-based large-area flexible PSCM Full size image Table 1 Parameters derived from the J-V curves of the champion rigid PSCs based on different SnO 2 substrates Full size table Furthermore, this potassium passivation strategy was employed for fabrication of the flexible PSCs. Figure 3d shows the champion J-V curves of the interface potassium passivated flexible PSCs based on low-temperature processed SnO 2 NCs. A comparable high efficiency device of 17.09% for RS and 17.18% for FS was obtained, with a high V oc of 1.095 V for RS and 1.090 V for FS, a J sc of 20.48 mA cm −2 for RS and 20.48 mA cm −2 for FS, and a FF of 0.76 for RS and 0.77 for FS, respectively. The corresponding EQE spectra is showed in Fig. 3e , which shows an integrated current density of 19.98 mA cm −2 . Figure 3f shows the 5 × 6 cm 2 large-area flexible PSCM based on low-temperature slot-die-coated SnO 2 NCs, which shows a competitive performance to the commercial Alfa–SnO 2 -based flexible PSCMs. The champion device shows a high PCE of 14.47% for RS and 14.89% for FS, with high V oc of 6.544 V for RS and 6.542 V for FS, J sc of 3.30 mA cm −2 for RS and 3.30 mA cm −2 for FS, and FF of 0.67 for RS and 0.69 for FS, respectively. Therefore, this interface potassium engineering is promising for hysteresis elimination and performance enhancement for low-temperature SnO 2 -based planar PSCs. Role of potassium ions at the interface Potassium ions have been added into PSCs and have shown an efficient passivation effect [29] , [36] . Recent reports attributed the passivation mechanism to the excess halides introduced by the additive of potassium iodide [36] , [37] . The excess halides passivate the vacancies and thereby inhibit the halide migration and suppress the non-radiative recombination [36] . However, for the KOH treatment carried out in this work, there is not excess halides introduced as the anion is OH − . To confirm that the interface engineering is performed by the K + ions instead of anions, we used a potassium acetate (KAc, KCH 3 COO) solution to treat the nanocrystalline SnO 2 interface and obtained the similar effect of hysteresis elimination (Supplementary Fig. 11 ). Thus, it is necessary to study the role of K ions at the interface. Interestingly, the K ions at the SnO 2 /perovskite interface has a great impact on the nucleation and growth of the perovskite films. When depositing the perovskite precursor onto different substrates without anti-solvent quench and annealing, we found large grains on low concentration potassium-treated substrate (Supplementary Fig. 12 ), but when a further increase of KOH on the surface of the substrate, too many nuclei formed, consuming too much solute to allow the nuclei to grow, and leading to small size grains in the final microstructure of the film. Therefore, an annealing-free porous film consisting of small size perovskite grains was found on the untreated SnO 2 ETL (PSK-NM) even after anti-solvent quench, but an annealing-free dense film with large grains formed on the KOH-treated SnO 2 ETL (PSK-KOH) film (Supplementary Fig. 13 ). Furthermore, after thermal annealing at 120 °C, the former showed a lot of PbI 2 crystals on the perovskite film surface, but the latter appeared a much clear and smooth surface with larger grains (Supplementary Fig. 14 ). The corresponding XRD result confirmed the residual PbI 2 in the annealed PSK-NM perovskite film (Fig. 4a ). It’s also noticed that before annealing the perovskite crystals in both samples showed a clear orientation of the (012) plane parallel to the substrate, but the preferential orientation disappeared after annealing (Fig. 4a ). Fig. 4 Properties of perovskite films with interface potassium passivation. a XRD patterns of different SnO 2 substrates-based perovskite films with or without thermal annealing. b A schematic of the perovskite growth process on different substrates. c UV-Vis spectra of different SnO 2 substrates-based perovskite films with/without thermal annealing. d The steady PL spectra of perovskites with/without interface potassium passivation. e The TRPL spectra of perovskites with and without interface potassium passivation. The inset plot shows the corresponding TRPL spectra when excitation laser is incident from the glass side. f Cross-section SEM image of the pristine perovskite device. g Cross-section SEM image of the perovskite device with interface potassium passivation Full size image Considering the strong ionic bond of KBr, it is possible that the K ions introduced from KOH could readily form KBr by substitutional reaction with the Br ions at the surface of the perovskite film [38] . The KBr − rich interface would passivate the halide vacancies at the interface to promote the high performance including the hysteresis elimination. Furthermore, the strong dipole of KBr would preferentially link PbX 2 and act as nucleus for perovskite formation, as proposed in Fig. 4b . The leaching of the Br − from the perovskite film then resulted in more I − rich perovskites to form, which is consistent with the red-shift of the UV-Vis spectra (Fig. 4c ), also confirmed by the EQE in the completed devices (Supplementary Fig. 7 ). In addition, the XRD also shows a slight shift to the lower angle (Supplementary Fig. 15 ), indicating the expansion of the lattice by incorporation of more I − in the crystal. This can also explain why the perovskite deposited on the KOH-treated ETL has much less free PbI 2 after annealing. The K + nucleus facilitate the perovskite crystal growth even without thermal annealing. Such annealing-free PSCs exhibit excellent photovoltaic performance of high PCEs of 18.16% for RS and 18.15% for FS, much higher than the non-treated device (11.74% for RS and 7.63% for FS) as shown in Supplementary Fig. 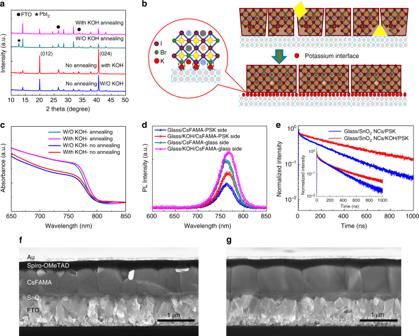Fig. 4 Properties of perovskite films with interface potassium passivation.aXRD patterns of different SnO2substrates-based perovskite films with or without thermal annealing.bA schematic of the perovskite growth process on different substrates.cUV-Vis spectra of different SnO2substrates-based perovskite films with/without thermal annealing.dThe steady PL spectra of perovskites with/without interface potassium passivation.eThe TRPL spectra of perovskites with and without interface potassium passivation. The inset plot shows the corresponding TRPL spectra when excitation laser is incident from the glass side.fCross-section SEM image of the pristine perovskite device.gCross-section SEM image of the perovskite device with interface potassium passivation 16 and Supplementary Table 4 . After the thermal annealing, the PSK-KOH perovskite shows a better quality, as revealed by the steady-state PL spectra (Fig. 4d ). Under the same excitation and detection conditions, the PSK-KOH perovskite has a stronger PL intensity than the PSK-NM perovskite, demonstrating the high quality of the whole perovskite film. This is further supported by time-resolved PL measurement using time correlated single photon counting (TCSPC) (Fig. 4e ). When the laser is incident from the perovskite side, the bottom ETL has a very little effect on the photogenerated carriers and thus the PL decay is dominated by the carrier recombination dynamics in the perovskite. The KOH-treated sample shows much longer lifetime, confirming relatively low non-radiative recombination of the perovskite. The cross-section SEM images (Fig. 4f, g ) show that in the normal direction of the film there is single-grain, which would promote the fast charge transport. When the excitation laser is incident from the glass side (the inset plots in Fig. 4e ), the KOH-treated ETL enhanced the interface charge extraction. Generally, in this case the PL decay is controlled by three components, bulk perovskite recombination, interface recombination through surface trapping and carrier extraction by ETL. It is reasonable to assume the interface recombination is not significant because of the corresponding high efficiency solar cells. To quantitatively describe this process, we have fit the PL decay curves by the two-exponential function. 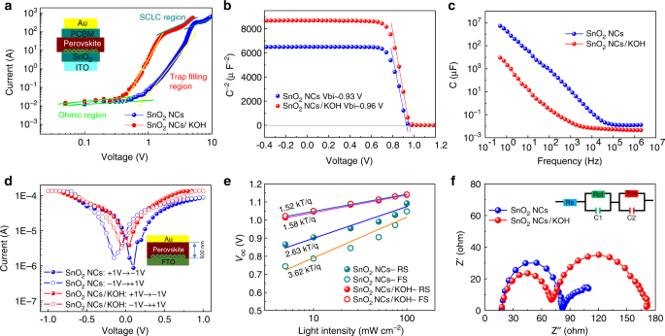Fig. 5 Mechanism analysis of interface potassium passivation.aDarkJ–Vcharacteristics of electron-only devices with and without interface potassium passivation. The inset shows the structure of the corresponding electron-only device.bMott–Schottky plots of PSCs with and without interface potassium passivation.cCapacitance–frequency plots of PSCs with and without interface potassium passivation.dThe logarithmicI-Vplots of the FTO/CsFAMA/Au and FTO/KOH/CsFAMA/Au device, respectively. The inset shows the structure of the corresponding device.eTheVocvs. Light Intensity curves of PSCs with and without interface potassium passivation andfthe typical Nyquist plots of PSCs with and without interface potassium passivation. The inset shows the equivalent circuit diagram Two PL decay curves are well fitted and the fitting parameters are listed in Supplementary Table 5 . The short time constant ( τ 1 ) can be ascribed to electron extraction. The shorter constant 12.02 ns is acquitted for the treated ETL, relative to the longer one in untreated ETL. It should note the weight of the faster component significantly increases from 35 to 45%, clearly indicating the enhanced electron extraction. The slow component ( τ 2 ) is ascribed to bulk recombination, significantly increased from 226.83 ns for untreated sample to 273.68 ns for treated sample, indicating the improved quality in perovskite by the KOH treatment. The perovskite also showed a lower surface potential difference with potassium passivation (Supplementary Fig. 17 ), therefore, the high quality of the perovskite along with the passivated traps at the interface would benefit the performance of the devices including the hysteresis [39] . Reduced defects at the interface for the reduced hysteresis In order to further explore the interface effects of potassium on the devices, the electron-only devices of a glass/FTO/SnO 2 /with or without KOH/perovskite/PCBM/Au architecture were fabricated for accurately assess the trap density in these different devices. The dark J–V characteristics were measured to obtain the electron densities for all these devices. Figure 5a shows the dark J–V curves of these electron-only devices with/without interface potassium treatment. The space-charge-limited-current (SCLC) technique was used to estimate the trap densities of these devices [40] , [41] . The linear region at low bias voltage reveals an ohmic-type response, and a marked increase of the current injection follow the increase of the bias voltage at the intermediate region is identified as the trap-filling process. The kink point between these two regions is defined as the trap-filling limit voltage ( V TFL ), and therefore the trap density ( N d ) in devices can be calculated from the following relation [41] : 
    V_TFL = eN_dL^2/2εε _0,
 where e presents the elementary charge, ε stands for the relative dielectric constant, ε 0 is the vacuum permittivity and L is the thickness of the perovskite films. The electron trap density in the potassium passivated device is calculated to be 4.42 × 10 15 cm −3 , which is much lower than that for the pristine device (8.86 × 10 15 cm −3 ). This reduced trap density can be attributed to the high quality of the perovskite crystals induced from the potassium passivation, which also contributes to reduced hysteresis in the PSCs. Fig. 5 Mechanism analysis of interface potassium passivation. a Dark J–V characteristics of electron-only devices with and without interface potassium passivation. The inset shows the structure of the corresponding electron-only device. b Mott–Schottky plots of PSCs with and without interface potassium passivation. c Capacitance–frequency plots of PSCs with and without interface potassium passivation. d The logarithmic I-V plots of the FTO/CsFAMA/Au and FTO/KOH/CsFAMA/Au device, respectively. The inset shows the structure of the corresponding device. e The V oc vs . Light Intensity curves of PSCs with and without interface potassium passivation and f the typical Nyquist plots of PSCs with and without interface potassium passivation. The inset shows the equivalent circuit diagram Full size image Figure 5b illustrates the Mott–Schottky (M-S) plots of these PSCs at 10 kHz. The interface engineered PSC demonstrates an increased build-in potential ( V bi ) of 0.96 V and a corresponding decreased carrier density ( N d ) of 1.01 × 10 16 cm −3 , compared with the non-treated solar cell (0.93 V and 1.18 × 10 16 cm −3 , respectively), which indicates fast charge collection and less carrier accumulation at the interface [42] , [43] , [44] . In addition, a capacitance–frequency ( C - f ) plots is also conducted as shown in Fig. 5c . Generally, the capacitance of the devices in the low-frequency regime may be ascribed to ionic migration to the contact interface [44] , [45] , [46] . The perovskite device with interface potassium treatment presents decreased capacitance compared with the pristine device, which in turn decreases the hysteresis of the device. Besides, we characterized the J - V properties by scanning from negative bias to positive bias, and then re-scan from positive bias to negative bias of these two perovskite films with/without potassium passivation. The device architecture is showed in Fig. 5d , and the corresponding logarithmic plots indicate the misalignment of the perovskite films under contrast sweep direction. A significant misalignment of the non-passivated perovskite films shows more moveable ions compared with the potassium passivate perovskite films. The change of the V oc of the PSCs made from the SnO 2 ETL with/without the KOH treatment was also measured under different light intensity (Fig. 5e ). It is found that a more monotonic increase in V oc with the light intensities under either RS or FS of the potassium passivated device compared with the non-passivated devices. As is well known, the deviation of the slope from unity kT / q (where k is the Boltzmann constant, T represents the absolute temperature and q denotes the elementary charge) suggests a trap-assisted recombination in solar cells [32] , [47] . The PSC with potassium interface passivation shows a slope of 1.52 kT / q , which is much lower than the non-passivated device (2.63 kT / q ) (Fig. 5e ). It indicates a substantially reduced trap-assisted recombination and efficient charge extraction resulting from suppressed recombination. This is also evident from the electrochemical impedance spectroscopy (EIS) measurement, a useful technique that reveals the potential carrier transport behaviours in the PSCs [48] , [49] , [50] . The Nyquist plots of these devices with interface passivation or non-passivation were obtained under AM 1.5 G sunlight illumination and with an applied bias voltage of 1.0 V close to the V oc as shown in Fig. 5f . There are two different semicircles which are located at different frequency ranges in the Nyquist plots. Generally, the high-frequency component is the signature of the charge transport resistance ( R ct ), and the low-frequency one corresponds to the charge recombination resistance ( R rec ) occurring at the interfaces [51] , [52] . The fitted R ct and R rec of these devices were plotted with the applied forward biases (Supplementary Fig. 18 ). The R ct value in the interface potassium passivated perovskite is decreased, while the R rec is much higher compared with the pristine one. Then the EIS data obviously shows the improved charge transport, as well as the reduced recombination in PSCs with interface potassium passivation. Conclusion In summary, we reviewed the recently reported works about the PSCs using various SnO 2 as the electron transporting materials and conclude that the hysteresis phenomenon is commonly observed in all these devices, except for additional treatments. Based on our analysis, we provided a facile interface passivation strategy with potassium treatments for SnO 2 ETLs to obtain high efficiency, hysteresis-free, stable and low temperature fabricated planar PSCs on glass and flexible PSCs as well as flexible PSCMs on plastics. We achieved an outstanding performance of rigid planar PSC with PCE of 20.50% for RS and 20.46% for FS and a flexible PSC with PCE of 17.09% for RS and 17.18% for FS on a small aperture area of 0.16 cm 2 after passivation, respectively. In addition, we also obtained a high PCE of 15.22% for a flexible PSCM based on slot-die-coated Alfa–SnO 2 substrate and a PCE of 14.89% for homemade SnO 2 NCs. The additional of the K ions in the interface forms KBr that thus passivates the surface defects of the perovskite to promote the high performance and hysteresis-free properties. The positive effects brought by the potassium ions are promising for pursuing high performance and stable large area PSCMs. This universal SnO 2 surface engineering strategy opens an effective way to fabricate the high quality SnO 2 ETL for the planar PSCs and PSCMs. Materials The SnO 2 colloidal dispersion (tin (IV) oxide, 15% in H 2 O colloidal dispersion) was purchased from Alfa Aesar. The SnCl 2 ·2H 2 O, SnCl 4 ·5H 2 O, anhydrous SnCl 4 solution and KOH were purchased from Aladdin. Lead iodide (PbI 2 ) and lead bromine (PbBr 2 ) were purchased from TCI. Formamidinium iodide (FAI) and methylammonium bromine (MABr) were purchased from Lumtec Technology Corp., Taiwan. The Spiro-OMeTAD was purchased from Xi’an Polymer Light Technology Corp. All other chemicals were purchased from Sigma-Aldrich or Alfa Aesar and used as received unless specified. Preparation of the rigid and flexible substrates The rigid FTO/glass or flexible ITO/PET substrates were first etched using a femtosecond laser machine. Then they were cleaned through ultrasonic cleaning by detergent, pure water, and ethyl alcohol for 20 min, respectively. After that, the dry-air gas flow was employed to dry the films and then treat the films by plasma for 5 min before use. Preparation of the SnO 2 films Alfa–SnO 2 films: The as purchased SnO 2 colloidal dispersion was diluted by water (1:3 wt), and then spin-coated onto the clean FTO/glass substrates at 3000 rpm for 30 s and repeated for two times, then annealed at 150 °C for 1 h. For flexible devices, the SnO 2 NCs/isopropanol solution was spin-coated onto the clean ITO/PET substrates, followed by the annealing at 140 °C for 1 h. Water Alfa–SnO 2 films: The diluted Alfa–SnO 2 solution was spin-coated on the bare glasses and sintered at 150 °C for 30 min. After cooling down, a proper amount of deionized water was added into a vessel to bath the as-sintered Alfa–SnO 2 /glasses for different time. SnO 2 NCs films: The SnO 2 NCs were achieved by a low temperature hydrothermal method. The anhydrous SnCl 4 solution was diluted to 0.15 M by iced deionized water, and then kept in an oven at 90 °C. After hydrothermal treatment for an hour, the solution was washed by diethyl ether/isopropanol mixed solution for three times and followed by centrifugal separation. The centrifuged solid was re-dissolved in isopropanol with a concentration of 10 mg mL −1 . Lastly, the SnO 2 NCs/isopropanol solution was spin-coated onto the clean FTO/glass substrates at 3000 rpm for 30 s and repeated for three times, then annealed at 180 °C for 1 h. For flexible devices, the SnO 2 NCs/isopropanol solution was spin-coated onto the clean ITO/PET substrates, followed by annealing at 140 °C for 1 h. Spin-coated SnO 2 films: The spin-coated SnO 2 films were fabricated using SnCl 4 •5H 2 O/isopropanol precursor. A 50 µL of 0.075 M SnCl 4 •5H 2 O/isopropanol precursor was spun onto the clean FTO/glass substrates at a spin rate of 3000 rpm for 30 s. The films were then annealed at 180 °C for 1 h. After cooling down, the as-sintered SnO 2 substrates were soaked into a hot water bathing at 90 °C for 1 h. Finally, the films were annealed at 180 °C for 30 min. CBD deposited SnO 2 films: The CBD–SnO 2 films were achieved by chemical bath deposition method. 5 g urea was firstly dissolved into 400 mL deionized water, followed by the addition of 100 µL thioglycollic acid and 5 mL HCl (37 wt%). Finally, the SnCl 2 ·2H 2 O powder was dissolved in the solution at a concentration of 0.012 M and then stored in fridge for 3 days before use. The as-cleaned FTO glass was soaked into the diluted SnCl 2 ·2H 2 O solution (0.002 M) for 2 h at 70 °C and then washed by deionized water and dried by gas gun blowing. The CBD process was repeated for three times in order to achieve the desired thickness, and followed by annealing at 180 °C for 1 h. KOH-treated SnO 2 films: The KOH powder was dissolved in water at a concentration of 5 mM, 10 mM, 20 mM, 50 mM and 100 mM respectively, and then spin-coated onto the SnO 2 films at 3000 rpm for 30 s, followed by annealing at 100 °C for 10 min. Slot-die-coated SnO 2 onto large area flexible plastic substrates: The SnO 2 films were deposited under ambient conditions using a homemade slot-die setup on a 3D mobile platform. The as-purchased Alfa–SnO 2 colloidal dispersion in water was diluted by H 2 O firstly, and then diluted using isopropanol (IPA), drop by drop, under continuous stirring, with the final volume ratio of H 2 O/IPA to 1:1. The diluted concentration was about 10 mg mL −1 , and the synthesized SnO 2 NCs were also diluted by isopropanol with a concentration about 10 mg mL −1 . The diluted SnO 2 solution was deposited on a clean ITO-PET substrate by slot-die coating for three cycles, followed by annealing at 140 °C for 1 h. The distance between substrate and slot-die lip was 0.25 mm ( Z = 0.25 mm). The coating speed was controlled by a built-in controller of the 3D mobile platform while the solution flow through the slot-die head was controlled by a syringe pump (stage speed V = 15 mm s −1 , the solution flow rate = 58 L s −1 ). Preparation of the mixed perovskite precursor The CsFAMA mixed perovskite precursor was prepared by dissolving 1.3 M organic cation (0.85 FAI and 0.15 MABr) and 1.4 M mixture of metal lead salts (0.85 PbI 2 and 0.15 PbBr 2 ) in a mixture solvent of DMF/DMSO (4:1, by volume), and then a 34 µL CsI solution (pre-dissolved as a 2 M stock solution in DMSO) was added to achieve the desired Cs 0.05 (FA 0.85 MA 0.15 ) 0.95 Pb(I 0.85 Br 0.15 ) 3 perovskite precursor solution with proper excess lead halide. Preparation of the Spiro-OMeTAD solution The Spiro-OMeTAD solution was prepared by firstly dissolving 73 mg Spiro-OMeTAD in 1 mL chlorobenzene. After that, 18 µL Li-TFSI (from 520 mg mL −1 stock acetonitrile solution) and 29 µL FK209 (300 mg mL −1 stock acetonitrile solution) and 30 µL 4-tert-butylpyridine, were added into the solution. The solution was continuously stirring for 10 min before use. Device fabrication The mixed perovskite precursor was spin-coated on these different SnO 2 substrates at a spin rate of 6000 rpm for 30 s with accelerated speed of 1000 rpm. At the last 5th second, a 100 µL green anti-solvent of ethyl acetate was drop-coated, and then the as deposited films were annealed at 120 °C for 45 min. After cooling down, the Spiro-OMeTAD solution was spin-coated on the perovskite films at 3000 rpm for 30 s. Finally, 80-nm thick of gold was deposited using thermal evaporation to complete the whole devices. The deposition of large area perovskite films was referred to a previous report [29] . First, a femtosecond laser was used to scribe the 5 × 6 cm 2 cleaned ITO/PET substrate to form the module substrate with six strips. Then different SnO 2 precursors were deposited on the cleaned module substrate via a slot-die coating method. The perovskite and Spiro-OMeTAD films were fabricated by spin-coating via the same procedure as the small devices except with more solvent dosage. Lastly, the device was laser-scratched again to form the series-connected module before deposition of the gold. Characterizations The SnO 2 nanoparticles were characterized using a high resolution TEM (Talos F200S, Thermo Fisher, USA). The surface morphologies and microstructures of SnO 2 films, perovskite films and the cross-sectional structure of these PSCs were investigated using a field-emission scanning electron microscopy (FESEM, Zeiss Ultra Plus). The SnO 2 and perovskite films were also characterized by TOF-SIMS (TOF.SIMS 5-100, ION-TOF GmbH), UV-Vis spectrometer (lambda 750 S, PerkinElmer), X-ray diffractometer (XRD, D8 Advance), atomic force microscope (AFM) and kelvin probe force microscope (KPFM) (SPM9700, Shimadzu, Japan), respectively. The thickness of the perovskite, SnO 2 and FTO tested in TOF-SIMS are approximately 500 nm, 100 nm and 800 nm, respectively. The EIS measurements of these PSCs were carried out by an EC-lab (SP300). The J - V curves of these PSCs were measured using a Keithley 2400 source meter at room environment. The light source was a solar simulator (Oriel 94023 A, 300 W) to match AM 1.5 G. The intensity of the light was 100 mW cm −2 calibrated by a standard silicon reference solar cell (Oriel, VLSI standards). All the devices were tested using a black metal aperture with a defined active area of 0.16 cm 2 for the small devices and 16.07 cm 2 for the large 5 cm × 6 cm PSCMs, respectively.